Suppression of population transport and control of exciton distributions by entangled photons Entangled photons provide an important tool for secure quantum communication, computing and lithography. Low intensity requirements for multi-photon processes make them idealy suited for minimizing damage in imaging applications. Here we show how their unique temporal and spectral features may be used in nonlinear spectroscopy to reveal properties of multiexcitons in chromophore aggregates. Simulations demostrate that they provide unique control tools for two-exciton states in the bacterial reaction centre of Blastochloris viridis . Population transport in the intermediate single-exciton manifold may be suppressed by the absorption of photon pairs with short entanglement time, thus allowing the manipulation of the distribution of two-exciton states. The quantum nature of the light is essential for achieving this degree of control, which cannot be reproduced by stochastic or chirped light. Classical light is fundamentally limited by the frequency-time uncertainty, whereas entangled photons have independent temporal and spectral characteristics not subjected to this uncertainty. Entangled quantum systems are known to outperform their classical counterparts in many applications such as quantum information processing [1] , [2] , quantum communication [3] , [4] , lithography [5] and metrology [6] . In addition, entangled light has promising opportunities as a novel spectroscopic tool [7] , [8] , [9] , [10] , [11] , [12] . This could be highly significant, as nonlinear spectroscopy has emerged as the most important tool for studying quantum dynamics in excitonic systems. For instance, 2D electronic spectroscopy with ultrashort pulses has been used to monitor energy transport processes [13] in photosynthetic complexes, but the broad bandwidth of the pulses prohibits selective excitation of a single excited state. Hence, typical spectra often contain many, overlapping features. Control over exciton distributions could help identify relaxation pathways by disentangling otherwise congested signals [14] , [15] . Such control is challenging: the electronic states of photosynthetic complexes form distinct manifolds with a fixed number of excitons, and the excitation of any two-exciton state can take place through many different intermediate single-exciton states. Interference between different excitation pathways further complicates the dynamics. Elaborate optimization techniques have been employed to enhance a certain pathway, which has to compete with rapid (femtosecond) population transport in the single-exciton manifold [16] . Entangled photons possess unique nonclassical spectral and temporal features, which predestine them as probes for the interaction between molecular excitations. The frequency-time entanglement of photon pairs offers novel control parameters, which can be used to manipulate population transport in the single-exciton manifold. Here, we examine two-exciton distributions created by the absorption of entangled photon pairs. Even though two-exciton states outnumber the single excitons, thus rendering optical signals even more complicated than classical signals of single excitons, they are worth investigating. They contain information on the many-body interactions between excitons, and on inter-exciton distances [17] . The respective two-exciton distributions can be detected by a variety of techniques, like two-photon absorption, fluorescence or two-photon counting. We present simulations of the bacterial reaction centre (RC) of Blastochloris viridis , depicted in Fig. 1a . Excitation energy transfer within the RC and the subsequent charge separation cascade convert the sunlight’s energy into a chemical potential gradient with near-unit efficiency [18] . Understanding the many-body physics of the bacterial RC could provide important insights for the construction of optoelectronic devices, which benefit from using the near-IR region of the solar spectrum [19] , [20] . Our model includes 12 single- e 1 , ···, e 12 and 41 two-exciton states f 1 ,··· , f 41 (for the labelling of states see the caption of Fig. 1 ), exciton transport is described by the Redfield equations (see Methods section). We aim to describe the excited state distribution induced by entangled light, which is different from the natural photosynthesis process [21] , [22] . 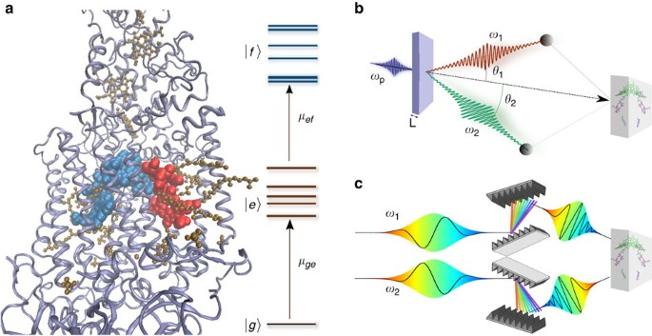Figure 1: Model system and proposed experimental setups. (a) The bacterial RC and its electronic level scheme. The active branch where charge separation takes place is shown in blue, the inactive in red. The model has 12e-states and 41f-states, labelled ase1,…,e12andf1,…,f41. (b) The proposed setup for entangled photons: a pump photon of frequencyωpis down-converted into two photons with frequenciesω1andω2, and directed onto the bacterial RC. We consider type-II down conversion, which means one of the photons is created along the ordinary axis of the crystal, and the other one along the extraordinary axis46. The different group velocities along these two axes create a time delay between the two-photon wavepacket—the entanglement timeT. Owing to energy conservation, the two photons are entangled in their frequenciesωp=ω1+ω2: both the green and red beam may have a very broad bandwidth, but as soon as the frequency of one of the two photons is measured, the wavefunction of the other beam collapses, and the frequency of the photon is sharply defined as well. By selecting the anglesθ1andθ2, one can tune the central frequencies of the entangled wavepackets. (c) The setup for chirped pulses: two laser pulses with frequenciesω1andω2are stretched in time by grating pairs in an anti-correlated manner, thus inducing frequency anti-correlations. Figure 1: Model system and proposed experimental setups. ( a ) The bacterial RC and its electronic level scheme. The active branch where charge separation takes place is shown in blue, the inactive in red. The model has 12 e -states and 41 f -states, labelled as e 1 ,…, e 12 and f 1 ,…, f 41 . ( b ) The proposed setup for entangled photons: a pump photon of frequency ω p is down-converted into two photons with frequencies ω 1 and ω 2 , and directed onto the bacterial RC. We consider type-II down conversion, which means one of the photons is created along the ordinary axis of the crystal, and the other one along the extraordinary axis [46] . The different group velocities along these two axes create a time delay between the two-photon wavepacket—the entanglement time T . Owing to energy conservation, the two photons are entangled in their frequencies ω p = ω 1 + ω 2 : both the green and red beam may have a very broad bandwidth, but as soon as the frequency of one of the two photons is measured, the wavefunction of the other beam collapses, and the frequency of the photon is sharply defined as well. By selecting the angles θ 1 and θ 2 , one can tune the central frequencies of the entangled wavepackets. ( c ) The setup for chirped pulses: two laser pulses with frequencies ω 1 and ω 2 are stretched in time by grating pairs in an anti-correlated manner, thus inducing frequency anti-correlations. Full size image Suppression of single-exciton transport Figure 1b depicts the proposed experimental setup. A photon of the pump pulse with frequency ω p is down-converted in a birefringent crystal into a pair of entangled photons with frequencies ω 1 and ω 2 . Energy conservation induces energy-time entanglement between the two photons, that is, the bandwidth of the pump pulse limits the width of the sum of the two photons’ frequencies. At the same time, different group velocities within the crystal can lead to a broad bandwidth of the individual photons, which may greatly exceed the one of their sum. This velocity delay can be characterized by the entanglement time T (ref. 23 ), which sets an upper bound on the time delay between the absorption of the two photons, and turns out to be decisive for the control of double-excitons. Entangled two-photon absorption has also been shown experimentally to be greatly enhanced compared with classical two-photon absorption [24] , thanks to its linear rather than quadratic scaling with the pump intensity [9] . By varying the entanglement time and the pump frequency, one can reveal the influence of exciton transport in the single-exciton manifold. If a peak becomes stronger with increasing T , this indicates that the intermediate state is populated by transport, and vice versa. This is illustrated by the population of the two-exciton state f 11 . It is depicted in Fig. 2a versus the pump frequency ω p and the entanglement time T , the total two-exciton population is normalized at every point, . This state is mostly excited through the single-exciton state e 5 , which in turn is populated directly by photon absorption as well as by transport. For long entanglement times, where effects of quantum light are diminished, there are a number of resonances between 22,000 and 24,000 cm −1 , for which f 11 is strongly excited. The resonance at ω p = ω f 11 =22,160 cm −1 stems from the direct excitation g → e 5 → f 11 , the others result from transport processes within the single-exciton manifold. As T is decreased, the additional resonances dissappear, and only the direct excitation pathway survives. As the entanglement time sets an upper bound on the time the system spends in the single-exciton manifold between the absorption of the first and the second photon, it can be used to minimize the influence of population transport. The same goal could also be attempted by using ultrashort classical laser pulses. However, the simultaneous high spectral resolution along the ω p axis is only made possible by the strong frequency entanglement between the two photons [11] , and cannot be realized with classical light. Even though each photon has a very broad bandwidth (see Supplementary Fig. S1 ), their sum is narrowly distributed. Hence, population transport can be suppressed by entangled photon absorption, and used to enhance the excitation of otherwise very weak states. In Fig. 2b , we repeat this calculation for state f 23 . This state is solely excited through the short-lived single-exciton state e 6 , which decays within 100 fs to state e 5 . The latter is in turn most strongly linked to f 11 . Thus, by varying the entanglement time, we can monitor how the e 6 → e 5 transport process decreases the f 23 -population and causes the simultaneous appearance of an additional resonance of f 11 at 24,000 cm −1 . In short, the selectivity along the ω p axis allows us to excite a distinct two-exciton state such as f 23 . Varying T then enables us to monitor transport processes in the subset of single excitons that are connected to the selected two-exciton state ( e 6 and f 23 in our case). Spectroscopy with ultrafast classical pulses cannot resolve specific single-exciton pathways. 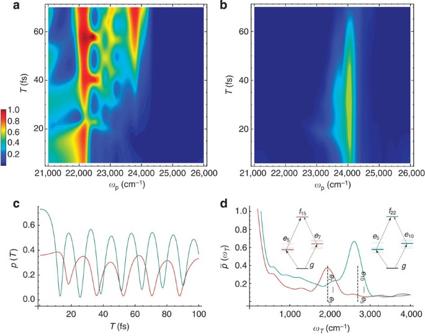Figure 2: Control of two-exciton distributions. (a) Variation of the population of statef11with the entanglement timeTand the central pump frequencyωp. Both beams have degenerate central frequenciesω1=ω2=ωp/2. (b) The same for statef23. (c) Population off15(red) forωp=22,600 cm−1andf22forωp=23,200 cm−1(red). (d) Fourier transform of (c). The insets depict the main excitation pathways leading tof15andf22. Figure 2: Control of two-exciton distributions. ( a ) Variation of the population of state f 11 with the entanglement time T and the central pump frequency ω p . Both beams have degenerate central frequencies ω 1 = ω 2 = ω p /2. ( b ) The same for state f 23 . ( c ) Population of f 15 (red) for ω p =22,600 cm −1 and f 22 for ω p =23,200 cm −1 (red). ( d ) Fourier transform of ( c ). The insets depict the main excitation pathways leading to f 15 and f 22 . Full size image Population oscillations reveal excitation pathways The evolution of f 11 also shows oscillations for some of the peaks with varying entanglement time. These oscillations shown in Fig. 2c are caused by the interference between excitation pathways. We observe strong oscillations, when ω p is tuned on resonance with f 15 ( f 22 ). State f 15 ( f 22 ) can be excited through the two intermediate states e 5 and e 7 ( e 10 ). As the excitation probability of any state is given by the coherent sum of all possible pathways leading to the state, this translates into a beating with the corresponding frequency difference ( Fig. 2d ). In contrast, the population of f 23 in Fig. 2b can only be excited through one intermediate state, and therefore shows no oscillations with T . Manipulating two-exciton distributions by quantum versus classical light We next discuss whether entanglement is essential for reaching the degree of control demonstrated above, and to what extent similar control could be achieved using properly shaped laser pulses. To achieve such control, we need to mimic both the suppression of single-exciton transport and the high-frequency resolution. Odd-order dispersion cancellation—an effect usually attributed to frequency entanglement—was demonstrated in Kaltenbaek et al . [25] using an ensemble of classical chirped laser pulses. To mimic the frequency entanglement by classical correlations, we consider pairs of chirped pulses as sketched in Fig. 1c . The frequency correlations are induced by opposite chirping (see Supplementary Fig. S2 for details). The chirped pulse parameters are adjusted to mimic the four-point correlation function of the entangled photons (equation (5)). In Fig. 3a , we compare the two-exciton distributions generated by entangled photon and by chirped pulses. The space between two lines corresponds to the fraction of a single state to the total population as a function of the pump frequency. This representation provides an intuitive picture of the degree of the control on the state distributions: When it rapidly varies with the pump frequency, one has a strong influence on the distribution by tuning this frequency. The two-exciton distributions in Fig. 3a are created by entangled pulses with high entanglement entropy [26] , whereas Fig. 3b shows low entanglement (details on the entanglement entropy are given in the Supplementary Note 1 ). In the first case, the entangled photons create exciton distributions that strongly depend on the pump frequency. Whenever an f -state is on resonance with the pump frequency, its excitation is enhanced. Similar features can be observed in the distributions created by chirped pulses. However, they now lie on top of a broad background caused by autocorrelation contributions 〈 E † E 〉 of the individual beams (see Supplementary Fig. S3 and Supplementary Note 2 ), which are absent for entangled photons. In order for these pulses to be sufficiently short to suppress single-exciton transport, they must have a very broad frequency spectrum, which creates this background. This difference is not apparent for a weakly entangled state (see Fig. 3b ) with low entanglement entropy. Both entangled photons and chirped pulses have lost their selectivity, and the populations look very similar to those produced by stochastic light. 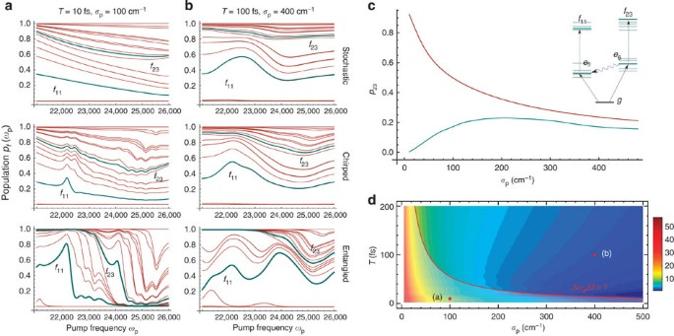Figure 3: Comparison with classical light and entanglement entropy. (a) Two-exciton state distributions induced by the absorption of entangled photon pairs (bottom), chirped pulses (middle) and stochastic light (top) withT=10 fs, andσp=100 cm−1. The central frequency of beam 2 is fixed atω2=11,000 cm−1, whileω1is varied. The two previously mentioned statesf11andf23are highlighted. (b) The same forT=100 fs, andσp=400 cm−1. (c) The population of statef23versus the pump bandwidthσpwithω1=11,908.3 cm−1andω2=12,200 cm−1. Population created by entangled photons is plotted in red, classical pulses in blue. (d) Entanglement entropy of the two-photon state (5) versus the entanglement timeTand the pump bandwidthσp. The area, for which (1) is violated, is separated by a red line, and the parameters of figures (a,b) are indicated. Figure 3: Comparison with classical light and entanglement entropy. ( a ) Two-exciton state distributions induced by the absorption of entangled photon pairs (bottom), chirped pulses (middle) and stochastic light (top) with T =10 fs, and σ p =100 cm −1 . The central frequency of beam 2 is fixed at ω 2 =11,000 cm −1 , while ω 1 is varied. The two previously mentioned states f 11 and f 23 are highlighted. ( b ) The same for T =100 fs, and σ p =400 cm −1 . ( c ) The population of state f 23 versus the pump bandwidth σ p with ω 1 =11,908.3 cm −1 and ω 2 =12,200 cm −1 . Population created by entangled photons is plotted in red, classical pulses in blue. ( d ) Entanglement entropy of the two-photon state (5) versus the entanglement time T and the pump bandwidth σ p . The area, for which (1) is violated, is separated by a red line, and the parameters of figures ( a , b ) are indicated. Full size image We recall that state f 23 is primarily excited via the short-lived state e 6 . Figure 3a demonstrates that one cannot selectively excite f 23 with chirped pulses. Owing to the large bandwidth of each beam, the autocorrelation contribution of the two beams excites brighter states with similar energies, such as f 22 and f 25 . We expect to be able to selectively excite this state by taking two laser beams, and tuning them on resonance with the g → e 6 and e 6 → f 23 transitions. In the following, we demonstrate that this may not be done as efficiently as with entangled photons. The population of f 23 induced by classical pulses with rectangularly shaped temporal envelope are compared with the population induced by entangled photons in Fig. 3c . We set ω 1 =11,908.3 cm −1 (the g → e 6 transition), and ω 2 =12,200 cm −1 (the e 6 → f 23 transition) as central frequencies of the two beams. Clearly, there is a trade-off between two competing mechanisms: pulses with a very narrow spectral density (that is, small σ p ) can better selectively excite a specific transition. However, as revealed by Fig. 3c , this only yields a small population in f 23 , as these pulses are longer, and the single-exciton transport depletes the intermediate state. Broadband (short) pulses (large σ p ) excite mostly brighter states around f 23 , and one ends up with a population of about 0.15 in f 23 for σ p =500 cm −1 . For an intermediate value σ p ∼ 200 cm −1 , we can achieve a slightly higher excitation of f 23 , but the population hardly exceeds 0.2. In marked contrast, the pump bandwidth of entangled photons does not influence the single-exciton transport, and we can reach a population of almost 0.8 with a spectrally narrow pump pulse. To explain our findings, we note that in order to control the excitation of a specific double-exciton state one seeks to minimize the time Δ t the system spends in the single-exciton manifold, and the sum frequency bandwidth Δ ω p . We use their product as a figure-of-merit for our degree of control. For classical pulses, we are fundamentally limited by the Fourier uncertainty, and , such that This explains why one cannot generate large populations of state f 23 by classical pulses. Moreover, one cannot violate equation 1 with chirped pulses either, as chirping can only increase the time-bandwidth product [27] , and equation 1 remains the lower bound. In the case of entangled photons in contrast, Δ t depends on the length of the crystal, that is, the entanglement time T , while Δ ω p is determined by the pump envelope. These are independent quantities, not Fourier conjugates, and their product has no lower bound. For the parameters of Fig. 3a , we have Δ t Δ ω p =0.18<<1. To discuss how this is related to the frequency entanglement of the two photons, we depict the entanglement entropy [26] of the entangled photon state versus T and pump bandwidth σ p in Fig. 3d . We also add the ‘classical boundary’ when Δ t Δ ω p =1. Clearly, whenever the entanglement entropy is large, one violates the inequality (1). Hence, strongly entangled photons clearly provide an advantage over classical light. The converse is not true, as a very short-entanglement time does not guarantee strong frequency anti-correlations, even though it may violate the inequality (1). In conclusion, we have shown that entangled photon pulses offer a unique degree of control on two-exciton distributions of molecular aggregates. Controlling population transport in the single-exciton manifold can better reveal excitation pathways in the RC. This advantage is most pronounced, when the entanglement entropy is also maximal as seen in Fig. 3d . Finally, we note that our findings can be applied to any excitonic system with a similar level structure such as quantum dots or carbon nanotubes [28] . The model system The model Hamiltonian is taken from Fingerhut and Mukamel [29] . Its construction is based on X-ray structural data for B. viridis (PDB code: 1PRC) [30] , excitation energies are taken from Won and Friesner [31] , and Förster couplings are calculated in the dipole approximation. Restricting the charge transfer states to the active branch of the RC (see Fig. 1a ), the model incorporates 12 single-exciton states (6 charge-separated states and 6 molecular excitations), which can form 41 two-excitons in the active branch of the RC. Excitons e 1 – e 4 are charge-separated states, whereas e 5 – e 10 are Frenkel type (all states are labelled with increasing energies). Exciton transport induced by coupling to the environment is described by secular Redfield equation [32] (for details of the Master equation, see the Supplementary Methods ). This level of theory ensures a physically acceptable evolution of the density matrix for arbitrary (positive) times. It cannot account for more subtle phenomena, such as population oscillations or memory effects [33] , [34] . However, the suppression of single-exciton transport reported here relies on beating the time scales of the single-exciton dynamics with the short entanglement time. The precise form of these dynamics is not vital for this arguement to hold, and should therefore not alter the physical picture. The coupling to the radiation field is described by a dipole Hamiltonian in the rotating wave approximation, where V ( t ) denotes the exciton annihilation operator, and E ( t ) the photon annihilihation operator. Both are taken in the interaction picture with respect to the matter and radiation field Hamiltonians. Two-exciton populations The leading-order contribution to the two-exciton populations p f =tr{| f ( t )〉〈 f ( t )| ρ ( t )} calculated perturbatively in the quantum light intensities is given by the loop diagram in Fig. 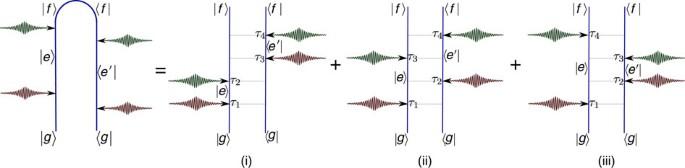Figure 4: Diagrammatic representation of the two-exciton states. Equation 3 is given by a single unrestricted loop diagram. It can be represented by the sum of fully time-ordered ladder diagrams (i)–(iii) (plus complex conjugated). The latter are necessary for a reduced description of an open quantum system. 4 , Figure 4: Diagrammatic representation of the two-exciton states. Equation 3 is given by a single unrestricted loop diagram. It can be represented by the sum of fully time-ordered ladder diagrams (i)–(iii) (plus complex conjugated). The latter are necessary for a reduced description of an open quantum system. Full size image with B f ( t )=| f ( t )〉〈 f ( t )|, Γ denotes the set of control parameters such as frequencies, pump envelopes and so on, and the time-ordering operator is represented by . In the figures we have normalized p f , such that ∑ f p f ( t ; Γ)=1 at each t . The electric field enters in (3) through the same four-point correlation function responsible for the Hong-Ou-Mandel dip [35] and other photon correlation effects, which is the reason we expect to see genuine entanglement effects in the present calculations. Additionally, the exciton system enters through the four-point correlation function, just like the photon echo and similar spectroscopic techniques. This is the reason it contains the same information as these conventional techniques. To obtain a reduced description where environmental degrees of freedom are eliminated, we need to break up the above equation into three fully time-ordered ladder diagrams as depicted in Fig. 4 (plus their complex conjugates). We evaluate the time integrations by recasting the field correlation function in the frequency domain which allows us to carry out the time integrations, resulting in equations (S25)–(S27) of the Supplementary Methods . The remaining integrations can be performed analytically using contour integrations (see Supplementary Methods for details). The final sum-over-states expressions are given by equations (S28)–(S30) of the Supplementary Methods . The twin photon state In Fig. 1b of the main text, we outline the proposed experimental setup: a pump pulse with central frequency ω p is down-converted in a birefingent crystal into two photons of frequencies ω 1 and ω 2 . In this situation the quantum state of light is described by the wavefunction [36] where the photon creation operator in the frequency mode ω and Φ( ω a , ω b ) is the two-photon amplitude, Here, A p ( ω )= A 0 /( ω – ω p + iσ p ) is the envelope of the pump pulse, and L the length of the birefringent crystal in the direction of the pulse. The two time scales T 1 =(1/ v p −1/ v 1 ) L and T 2 =(1/ v p −1/ v 2 ) L represent the time delays aquired between the various beams in the course of the propagation through the crystal. Here, v denotes the group velocity of the pump pulse, or beams 1 and 2, respectively [37] , [38] , [39] , [40] . The two times T 1 and T 2 in equation 6 can be combined into the entanglement time T = T 2 – T 1 (ref. 23 ). Even though T does not show up directly in (6), it still turns out to be crucial for the behaviour of the correlation function. It sets an upper bound on the time between two successive interactions with the entangled photons. In this paper, we consider entanglement times on the order of 10–100 fs. The crystal length corresponding to these times depends on the birefringent crystal in use; for instance, in the case of a BBO crystal, this corresponds to crystal lengths between 50 and 500 μm [41] , which have been used experimentally [42] . Pulse shaping [43] can be used to further control the beams. As a direct consequence of this state, the four-point correlation function in equation 3 factorizes into two parts 〈 E † ( ω ′ a ) E † ( ω ′ b ) E ( ω b ) E ( ω a )〉=Φ * ( ω ′ a , ω ′ b )Φ( ω a , ω b ). Classical light Exciton distributions can be manipulated by classical frequency correlations. Recently, several effects, for example, dispersion cancellation [25] and ghost imaging [44] , [45] , that were thought to be genuine quantum effects have been demonstrated by classical light. In order to establish the impact of genuine frequency quantum entanglement (as opposed to classical frequency correlations) on the exciton distributions, we need to mimic the frequency entanglement of twin photons by classical frequency correlations. The heuristic models for chirped pulses and the stochastic light are designed to reproduce the two-point (〈 E † ( ω ) E ( ω ′)〉) (see Supplementary Fig. S3 ) as well as the four-point correlation function (〈 E † ( ω ′ a ) E † ( ω ′ b ) E ( ω b ) E ( ω a )〉) of the entangled photons, details are given in Supplementary Fig. S3 and Supplementary Note 2 . Assuming rectangularly shaped pulses in time domain, we further use for the laser pulses in Fig. 3 How to cite this article: Schlawin, F. et al . Suppression of population transport and control of exciton distributions by entangled photons. Nat. Commun. 4:1782 doi: 10.1038/ncomms2802 (2013).